Nitroalkanes as thioacyl equivalents to access thioamides and thiopeptides Thioamides are an important, but a largely underexplored class of amide bioisostere in peptides. Replacement of oxoamide units with thioamides in peptide therapeutics is a valuable tactic to improve biological activity and resistance to enzymatic hydrolysis. This tactic, however, has been hampered by insufficient methods to introduce thioamide bonds into peptide or protein backbones in a site-specific and stereo-retentive fashion. In this work, we developed an efficient and mild thioacylation method to react nitroalkanes with amines directly in the presence of elemental sulfur and sodium sulfide to form a diverse range of thioamides in high yields. Notably, this convenient method can be employed for the controlled thioamide coupling of multifunctionalized peptides without epimerization of stereocenters, including the late stage thioacylation of advanced compounds of biological and medicinal interest. Experimental interrogation of postulated mechanisms currently supports the intermediacy of thioacyl species. Peptides have emerged as promising drug modalities and offer a number of advantages over small molecule drugs, including simpler design, straightforward synthesis, decreased immunogenicity, enhanced tissue penetration, and the ability to interact with underexplored targets [1] . However, their relatively short plasma half-life and low uptake by cells often limit their direct translation to the clinic [2] . Chemical modifications are frequently required to improve the ability of peptides to resist enzymatic degradation and to increase the pharmacological or drug-like properties [3] . The thioamide is the closest isostere of an amide with the same number of atoms, bond planarity, 3D shape and similar electronic properties. Nevertheless, the single-atom substitution of O to S renders intriguing chemical properties of thioamides over those of oxoamides, including unique thermodynamics [4] , enhanced conformational rigidity [4] , [5] , improved proteolytic stability [6] , and characteristic spectroscopic profiles [7] . Due to these subtle but profound changes, the thioamidation of biologically active peptides, although often difficult to realize synthetically, is highly desirable by medicinal chemists to improve the thermal/proteolytic stability and the pharmacokinetic properties of amide-containing drug candidates. For example, N -cyclohexylethyl-ETAV, a plasma-stable and cell-permeable inhibitor, with a site-incorporated thioamide in the backbone, gave a 28-fold extended metabolic period in human blood than its oxoamide counterpart (Fig. 1a ) [8] . Also the thioamidation of phenylpropionamide of the cyclic peptide anticancer cilengitide gave remarkable stability to thioamidated macrocyclic peptides in human serum (half-life 2160 min.) as compared to the all-oxo variant (half-life 540 min.) [5] . In nature, thioamides are accessed via various biosynthesis pathways to produce mono- to multiply-substituted thioamidated peptides with diverse biological properties [9] . Saalfelduracin A, for example, is a 26-membered cyclopeptide synthesized ribosomally that is post-translationally modified via Thz11-Thr12 as a thiopeptide by a drug-resistant gram-positive pathogenic bacterium, which profoundly increases its antibacterial activity (16 times higher than its oxoamide family member Saalfelduracin D) [10] . Fig. 1: Synthetic approaches to bioactive thioamides. a Examples and importance of thioamide moieties in bioactive compounds. b and c Current strategies and common limitations for thioamide synthesis. b An O → S exchange approach requires the use of excess sulfur reagents. c A multi-step sulfur incorporation approach to making thioacylating substrates to generate thioamides. d This work : A direct and general method to thioacylate amines with nitroalkanes using elemental sulfur. Full size image Although plagued by poor regioselectivity, chemoselectivity and yield issues, thioamide-containing peptides are traditionally synthesized by the conversion of oxoamides into thioamides, often by replacing O by S with the use of noxious and odorous thionating agents (Fig. 1b ) [11] , [12] , [13] . Alternatively, thioacylating fragments of the C -terminus of the peptide with preinstalled thiocarbonyl groups need to be prepared over multiple steps prior to the attachment of the N -terminus peptide amines (Fig. 1c ). Such thioacylating fragments are either synthesized from the activation of acids, followed by replacing O by S with Lawesson-based thionating reagents (Fig. 1c , up) [14] , [15] , [16] , [17] , [18] , or by the conversion of carboxylic acids into thioacids and then treatment with stoichiometric activating reagents (Fig. 1c , down) [19] , [20] , [21] . These strategies often resort to the use of excess activating reagents and suffer from practical difficulties on the bench, thereby limiting substrate scope and control. Nitroalkanes of various complexities are readily available building blocks for synthesis. For instance, there is a wide variety of catalytic asymmetric methods for the direct preparation of α -chiral nitroalkanes from commercially available nitromethanes by reaction with imines, aldehydes, and so forth [22] , [23] , [24] . In particular, primary nitroalkanes are widely used to synthesize carboxylic acids, which was first reported by Kornblum in 1956 [25] , [26] and later advanced by Mioskowski in 1997 [27] . In 2010, Johnston and coworkers pioneered the concept of umpolung amide synthesis (UmAS) via the oxidative coupling of α -bromo nitroalkanes with amines in the presence of N -iodosuccinimide and potassium carbonate [28] . The Johnston group further expanded their UmAS concept to an extensive range of chiral nitroalkanes and amines [29] , [30] , [31] , [32] , [33] , [34] . Inspired by this body of work and our own amidation studies with the Hayashi group [35] , we herein show the synergistic combination of readily available chiral nitroalkanes with amines and elemental sulfur provides a direct and efficient method to form thioamides and thiopeptides in excellent yields (Fig. 1d ). This one-pot thioamidation method effectively solves the multiple selectivity problems encountered when using Lawesson-type reagents and circumvents several practical complications in current synthetic sequences to activated thioacyl precursors. 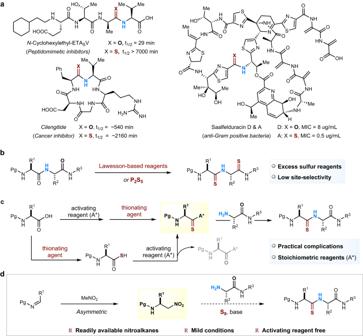Fig. 1: Synthetic approaches to bioactive thioamides. aExamples and importance of thioamide moieties in bioactive compounds.bandcCurrent strategies and common limitations for thioamide synthesis.bAn O → S exchange approach requires the use of excess sulfur reagents.cA multi-step sulfur incorporation approach to making thioacylating substrates to generate thioamides.dThis work: A direct and general method to thioacylate amines with nitroalkanes using elemental sulfur. Reaction discovery and optimization Our study began by exploring the reaction of the primary nitroalkane 1a with 3-phenylpropanolamine 2a in THF in the presence of K 2 CO 3 , where elementary S 8 was selected as the source of sulfur due to its low price, facile manipulation, and odorless nature (Table 1 , entry 1). These conditions gave the desired thioamide 4a in 37% isolated yield. Varying the base demonstrated Na 2 S (entry 4) to give superior yields of thioamide 3a over inorganic bases such as Na 2 CO 3 , Cs 2 CO 3 or K 2 CO 3 (cf. entries 1–3 and entry 4). Soluble nitrogen bases such as DBU, Et 3 N, pyridine was also found to be inferior to Na 2 S (cf. entry 4 and entries 5–7, Supplementary Table 1 for detailed optimization of solvent). No extra base gave thioamide 3a in low yield (12%) due to the amine 2a acting as a base, not as a reactant (entry 8). Although other electrophilic sulfur species were found to give comparably good yields (entries 9−12), elemental sulfur S 8 (2.0 equiv.) with Na 2 S (2.0 equiv.) stood out to afford 4a in excellent yield and operational convenience (entry 4). Table 1 Optimization of thioamide synthesis by reacting nitroalkanes with various sulfur sources a Full size table Substrate scope With optimized conditions identified, the substrate scope of various primary and secondary amines was investigated with the nitroalkane 1a (R 1 = CH 2 CH 2 Ph; Fig. 2a ). Primary amines carrying aliphatic, aromatic, alcohol, and alkene units were tolerated well under the reaction conditions, providing the thioamides 4a – 4e in high yields. Notably, besides secondary amines reacting efficiently ( 4f – 4h ), the stereo-integrities of the α-positions of chiral primary amines were retained without racemization, giving the thioamides 4j – 4l in good yields. When primary nitroalkanes bearing valuable functionalities such as –OH, –CO 2 Me, –Cl, and acetal were used, the corresponding thioamides 5a – 5m formed efficiently (Fig. 2b ). Besides nitromethane giving quick access to thioformamide 5h , nitroalkyl compounds bearing α-functionality smoothly furnished thioamides 5i – 5m . Subsequently, we applied this method to prepare thioamide pharmaceuticals and their analogues (Fig. 2c ). Examples include a selective σ1 agonist [36] analogue 6a , a transcriptional antiestrogen [37] S -analogue 6b , a late-stage functionalized antidepressive drug, amoxapine 6c , a ciprofloxacin alogue 6d , which were all synthesized in good yields. Such late-stage functionalizations of either primary or secondary amine positions clearly adds value to medicinal or chemical biology pursuits and readily allows for the thioamide diversification of chemical libraries from advanced intermediates. Fig. 2: Substrate scope and synthetic utility of the thioacylation of amines with nitroalkanes. Reaction conditions: Nitroalkane 1 (0.2 mmol), amine 2 (0.4 mmol), S 8 (0.4 mmol), Na 2 S (0.4 mmol), THF (2 mL), 24 h, rt; a Use of primary, secondary, and α-chiral amines. b Use of multifunctionalized nitroalkanes. c Late-stage thioacylation of bioactive substrates. Full size image Having established the general synthetic utility of the thioamidation method, we set out to synthesize more complex thiopeptides using readily available α-chiral nitroalkanes ( 7 ) [38] , [39] , [40] , [41] and α-amino ester-terminated fragments. Under the basic conditions of Na 2 S and S 8 at room temperature, the nitroalkane ( R )- 7a (ee > 99%) and 3-phenylpropylamine 2a formed the desired thioamide 8a in 96% yield and 76% ee, indicating partial epimerization over the reaction time (Fig. 3 , entry 1, column 2). Further studies indicated that the reaction temperature and the sulfur reagent critically affected the epimerization and chemical yield during the thioamidation process (Fig. 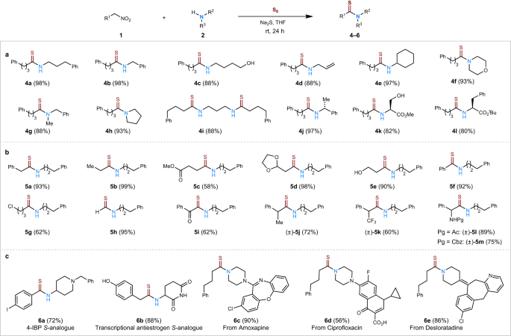Fig. 2: Substrate scope and synthetic utility of the thioacylation of amines with nitroalkanes. Reaction conditions: Nitroalkane1(0.2 mmol), amine2(0.4 mmol), S8(0.4 mmol), Na2S (0.4 mmol), THF (2 mL), 24 h, rt;aUse of primary, secondary, and α-chiral amines.bUse of multifunctionalized nitroalkanes.cLate-stage thioacylation of bioactive substrates. 3 , see Supplementary Table 2 optimization of sulfur reagent and temperature). When elemental S 8 was used as the sulfur source, the enantioselectivity of 8a dramatically increased but the chemical yield decreased as the temperature was lowered. When S 8 was changed to the disulfide 3d , the enantioselectivity improved at lower temperatures whilst keeping yields high. Optimal conditions were found over 36 h with the sulfur reagent 3d and Na 2 S in THF at −10 °C (Fig. 3 , entry 2, column 3). Here, enantiomerically pure nitroalkane ( R )- 7a (99% ee) and 3-phenylpropylamine 2a coupled to produce the desired thioamide 8a in 81% yield with no loss of stereogenic integrity. Fig. 3: Effect of temperature and sulfur (S) source on the stereogenicity of 8a. Reactions carried out with 0.1 mmol of 7a , 0.2 mmol of 2a , 0.2 mmol of S source and 0.2 mmol of Na 2 S in 1 mL of THF. Yield of isolated product. The ee value was determined by chiral-phase HPLC. Full size image With optimal conditions in hand for more complex substrates, the coupling of α-chiral nitroalkanes ( R )- 7 with a range of α-amino acid esters were screened (Fig. 4 ). This provided a significant level of generality and stereoselectivity without resultant epimerization of the thiopeptide products ( 10 – 11 ). Of note is the efficient coupling of sterically hindered secondary amines like proline ( 10u ) and the use of unprotected side chains for serine, tyrosine, tryptophan, and histidine ( 10p / j / l / q ). In addition, L -valine, L -Leucine, L -phenylalanine and the unnatural amino acid L -cyclohexyl glycine also couple readily with the L -tyrosine tert -butyl ester to afford thiopeptides 10v – 10x in good yields. (Fig. 4a ) Furthermore, the α-chiral nitroalkane ( R )- 7 (R 1 = CH 2 CH 2 Ph) reacted well with an amino dipeptide to produce the non-proteogenic tripeptide 11a in excellent diastereoselectively under these thioamidation conditions. Thioamide coupling between previously prepared tripeptide nitro-compounds and commercial amino acid esters also took place smoothly to afford the tetrapeptides 11b and 11c , bearing non-proteogenic residue groups, in moderate yields (Fig. 4b ). 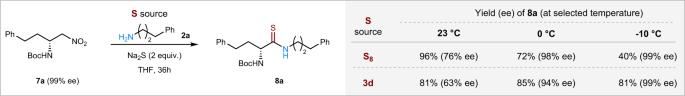Fig. 3: Effect of temperature and sulfur (S) source on the stereogenicity of 8a. Reactions carried out with 0.1 mmol of7a, 0.2 mmol of2a, 0.2 mmol of S source and 0.2 mmol of Na2S in 1 mL of THF. Yield of isolated product. The ee value was determined by chiral-phase HPLC. In practice, 11b could also be prepared in similar yields in DMF or DMF/THF mixtures, which is especially useful for substrates that are poorly soluble in THF (Supplementary Table 3 ). In addition, a dipeptide nitroalkane was prepared, which not only coupled very well with the lysine amine of pal-tripeptide-1 to give 11d in 73% yield, but also with an NH 2 -tetrapeptide to give the hexapeptide 11e in moderate yield. Unnatural α-aryl amino esters, although form thioamides under our current conditions, they partially racemize even at very low temperatures, as illustrated with ( R )-phenyl glycine and amine 2a giving thioamide 8b . To further demonstrate the synthetic potential of this thioamidation method, a quick and convergent synthesis of closthioamide, a highly potent natural antibiotic featuring six thioamide bonds [42] , was achieved (Fig. 4c ). The synthesis was accomplished in a straightforward manner from nitroalkanes 12 and 15 and propane-1,3-diamine by iterative dual thioamidations over 6 steps in 30% overall yield. Taken together, this method to form thioamide bonds provides a conceptually and reliable way to construct diverse thiocarbonyl polypeptides with no loss of stereogenic integrity and strategically allows ready preparation of mixed oxo/thioamide congeners of bioactive natural product and medicinal leads. Fig. 4: General synthesis of D / L -thiopeptides from unnatural nitroalkane ( D ) precursors and L -amino acids. Reaction conditions: 10a (0.1 mmol), 11a (0.2 mmol), Na 2 S (0.2 mmol), 3d (0.2 mmol) in THF (1 mL), stirred at −10 °C for 36 h. Isolated yields are given in brackets. a Scope of thiopeptide bond formation. b Example of thioamide-substituted peptides. 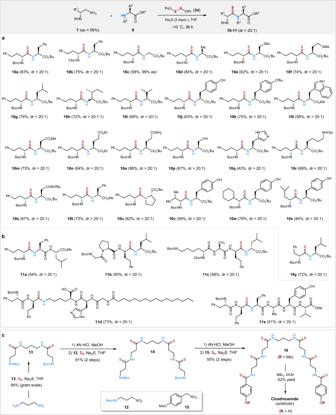Fig. 4: General synthesis ofD/L-thiopeptides from unnatural nitroalkane (D) precursors andL-amino acids. Reaction conditions:10a(0.1 mmol),11a(0.2 mmol), Na2S (0.2 mmol),3d(0.2 mmol) in THF (1 mL), stirred at −10 °C for 36 h. Isolated yields are given in brackets.aScope of thiopeptide bond formation.bExample of thioamide-substituted peptides.cTotal synthesis of closthioamide. c Total synthesis of closthioamide. Full size image Mechanistic studies We next turned our attention to shedding light on the reaction mechanism (Fig. 5 ). Based on our observations and literature reports [43] , [44] , [45] , [46] , [47] , there are three plausible mechanistic pathways to form thioamides from primary nitroalkanes and amines in the presence of electrophilic sulfur sources. One possibility is that the primary nitroalkane reacts with the amine and generates an oxoamide 17 first [31] , [35] , which is then converted into its thioamide 4a by the sulfur reagents (Fig. 5a , Path A). However, when the pre-made amide 17a was exposed to our standard reaction conditions, no thioamide 4a was observed and only the oxoamide 17a was recovered (Fig. 5b ). Also, when pre-formed amide 17a and primary nitroalkane 1a and 1-butylamine were exposed to our standard reaction conditions, only the amide 17a and the thioamide product 4l were identified and isolated (no mixed thioamides were detected). These reactions clearly rule out oxoamide formation prior to thioamide formation. Another possibility is that the amine reacts with electrophilic source of sulfur and generates an electrophilic amine species such as 18 (Fig. 5a , Path B) [28] . This electrophile then reacts with nitroalkane 1 in the presence of base to generate an α-amino nitroalkane 19 , which further reacts with sulfur species to afford thioamide 4 . To test this possibility, the sulfur amine 18a was premade and treated with the sodium salt of 1b , but no reaction was observed (Fig. 5c ). In addition, the proposed α-amino nitroalkane 19a was pre-made via a reported procedure [44] and was treated to the thioamidation conditions and no thioamide 21 was detected, only the starting nitroalkane 19a was recovered. As a third possibility, the nitroalkane reacts with the sulfur reagents and generates a thiocarbonyl intermediate 20 in situ, which is subsequently trapped with amine to generate the thioamide product 4 (Fig. 5a , Path C). To interrogate this mechanistic possibility (Fig. 5d ), the nitroalkane 22 was mixed with Na 2 S and S 8 in DMSO-d 6 for NMR and HRMS studies (Reactions (5)). Here, we observed the conversion of nitroalkane 22 to the dithiocarboxylate 23 . In addition, the nitroalkane 24 bearing a free γ-alcohol group was reacted with S 8 and Na 2 S, either in the presence or absence of external nucleophiles (cf. Reactions (6) and (7)). Both cases gave the thiolactone 25 . These experiments imply the intermediacy of a reactive thioacyl species like 20 , which NO 2 leaving group as supported by ion chromatographic analysis on crude reaction mixtures, for example, a 91% yield of nitrite salts was formed between nitroalkane 1a and amine 2a under standard reaction conditions (Supplementary Fig. 6 ). Fig. 5: Experimental studies to interrogate plausible reaction pathways and intermediates to form thioamides under S 8 /Na 2 S-based conditions. a Possible mechanistic pathways for the formation of thioamides from primary nitroalkanes and amines. b Control reactions to interrogate Path A. c Control reactions to interrogate Path B. d Control reactions to trap proposed thioacyl intermediate 20 in Path C. e Control reaction for the formation of thioacyl intermediate 20 . f Proposed reaction pathway in the conversion of primary nitroalkanes to thioamides via thioacylating species 20 . Full size image Having gained experimental evidence to support a putative thioacyl intermediate 20 , further control reactions were carried out to shed light on plausible intermediates prior to thiocarbonyl generation (Fig. 5e ). First, Na 2 S is considered to react with the starting nitroalkane to generate the α-carbanion/aci-nitronate sodium salt of 1a in high concentrations. We therefore used the pre-formed Na + salt of 1a to test its reaction with the amine 2a in the presence of Na 2 S/S 8 either under air or under Ar. Both cases gave the desired thioamide 4a in 80% yield (see Reaction (8)). Second, the pre-formed Na + salt of 1a when treated with amine 2a and Na 2 S in the absence of S 8 did not proceed at all. In the absence of Na 2 S, treatment of the pre-formed Na + salt of 1a with amine and S 8 formed the thioamide very slowly (see Reaction (9) and Reaction (10)). These results indicate that both S 8 and Na 2 S are required for a productive thioamidation process. Third, the β-cyclopropyl nitroalkane 27 was prepared as its pure cis -isomer for radical clock experiments to determine whether carbon-centered radicals form α to the nitro group [45] , [46] , [47] . In the event, when cis - 27 was reacted with the amine 2a in the presence of Na 2 S and S 8 , it generated the cis -thioamide 28 exclusively in moderate yield (Reaction (11)), thereby providing evidence that α-carbon radicals do not form (Supplementary Fig. 8 ). Based on the above control experiments, a general mechanism for this mild and direct thioamidation reaction is proposed in Fig. 5f . It is known that elemental sulfur can be activated by Na 2 S to produce S 3 radical anions [48] , [49] , which are expected to be the key reactive species in the thioamidation process. Indeed, further control reactions and EPR experiments (Supplementary Fig. 10 ) suggested the temperature-dependent formation of S 3 radical anions when using either S 8 or the disulfide 3d , thus indicating the reaction with 3d /Na 2 S systems follows a similar mechanism to that given in Fig. 5f (cf. 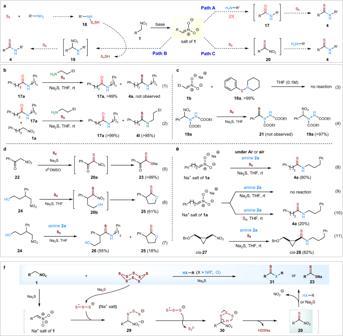Fig. 5: Experimental studies to interrogate plausible reaction pathways and intermediates to form thioamides under S8/Na2S-based conditions. aPossible mechanistic pathways for the formation of thioamides from primary nitroalkanes and amines.bControl reactions to interrogate Path A.cControl reactions to interrogate Path B.dControl reactions to trap proposed thioacyl intermediate20in Path C.eControl reaction for the formation of thioacyl intermediate20.fProposed reaction pathway in the conversion of primary nitroalkanes to thioamides via thioacylating species20. Supplementary Table 5 , Supplementary Fig. 11 ). Thus, the sodium salt of 1 , generated in situ by deprotonation with Na 2 S, couples with a S 3 radical anion at the α-carbanion position to afford a radical dianion salt 29 , which is oxidized by another S 3 radical anion to generate the organotrisulfide 30 [50] , [51] , [52] , [53] . Subsequent β-elimination of intermediate 30 then generates the thioacylating species 20 that can be captured by a suitable nucleophile to afford the product 31 or 23 . Although beyond the scope of this initial disclosure, our current studies do not discount other pathways to the formation of putative α-thio nitroalkanes like 30 and thioacyl species like 20 , including UmAS-based rationales. In conclusion, the reaction method described herein is the general method to efficiently access thioamides and thiopeptides from readily available nitroalkanes and amines. The method is straightforward in operation, chemoselective in functional group tolerance, stereochemically robust to potentially epimerizable substrates and products, and avoids extensive protection and deprotection procedures. In addition, the use of commercial or readily synthesized chiral nitroalkanes as masked thioacylating agents establishes a practical alternative to the longstanding reliance of carboxylic acid feedstocks in thiopeptide chemistry. A wide range of chiral primary nitroalkanes can be readily prepared in enantiopure form through reliable asymmetric methods, which renders this methodology relatively practical for complex systems. The use of nitroalkanes as formal equivalents to activated thiocarbonyl groups now provides a general means to make thio-based value-added compounds and targeted chemical libraries, even beyond peptide chemistry. The application of this current method in the solid phase synthesis of thioamide-containing peptides is ongoing in our group and will be published in due course. General thioamide coupling procedure With no special precautions from air or water, the nitro compound 1 (0.2 mmol) is added to a 10 mL reaction tube, followed by the sequential addition of THF (2 mL), S 8 (2.0 equiv. ), Na 2 S (2.0 equiv.) and the amine 2 (2.0 equiv.). The reaction is monitored by TLC until the nitroalkane appears consumed, typically after 24 h, after which the reaction is quenched with sat . NH 4 Cl, extracted with ethyl acetate, and the organic phases collected and dried over anhydrous Na 2 SO 4 . After filtration, the solution is concentrated under reduced pressure and the crude residue purified by silica-gel flash-column chromatography. General thiopeptide coupling procedure The chiral β-amino nitro compound 7 (0.1 mmol) is added to a 10 mL reaction tube, followed by the addition of THF (1 mL) and cooled down to −10 °C, after which Na 2 S (2.0 equiv., 0.2 mmol), 3d (2.0 equiv.) and the amine 9 (2.0 equiv.) are added with stirring. The reaction is monitored by TLC until complete, typically within 36 h, quenched with sat . NH 4 Cl, and the crude product extracted with ethyl acetate. After the organic phases are collected, dried over anhydrous Na 2 SO 4 and filtered, the solution is concentrated under reduced pressure and the crude product purified by silica-gel flash-column chromatography.